Revealing the properties of Mn2Au for antiferromagnetic spintronics The continuous reduction in size of spintronic devices requires the development of structures, which are insensitive to parasitic external magnetic fields, while preserving the magnetoresistive signals of existing systems based on giant or tunnel magnetoresistance. This could be obtained in tunnel anisotropic magnetoresistance structures incorporating an antiferromagnetic, instead of a ferromagnetic, material. To turn this promising concept into real devices, new magnetic materials with large spin-orbit effects must be identified. Here we demonstrate that Mn 2 Au is not a Pauli paramagnet as hitherto believed but an antiferromagnet with Mn moments of ~4 μ B . The particularly large strength of the exchange interactions leads to an extrapolated Néel temperature well above 1,000 K, so that ground-state magnetic properties are essentially preserved up to room temperature and above. Combined with the existence of a significant in-plane anisotropy, this makes Mn 2 Au the most promising material for antiferromagnetic spintronics identified so far. In a stack including a magnetically ordered material, tunnel anisotropic magnetoresistance (TAMR) represents the variation of resistance across a tunnel barrier, as a function of the angle between the direction of the moments and that of the current (or with respect to a crystallographic direction) [1] , [2] . A condition for large TAMR is the presence of large spin-orbit (SO) coupling. Magnetoresistive effects in excess of 10% have been obtained with Co/Pt ferromagnetic bilayers, where the SO interaction essentially arises from the noble Pt atoms [2] . The number of ferromagnetic alloys between 3 d transition metals and noble metals is relatively small, however. The fact that TAMR devices may incorporate an antiferromagnetic (AFM) layer instead of a ferromagnetic one could be exploited in novel spintronic devices [3] . AFM materials being largely insensitive to the effect of an external magnetic field, the parasitic fields that may affect Giant Magnetoresistance (GMR) or Tunnel Magnetoresistance (TMR) nanodevices would not affect TAMR devices. This has stimulated the search for AFM alloys combining high Néel temperature ( T N ) and large SO coupling effects [4] , [5] . Low-temperature ( T ) magnetoresistive effects in excess of 100% have been obtained in TAMR stacks incorporating AFM MnIr [6] . Mn alloys containing noble metals are often AFM [7] , [8] . However, this has not been considered to be the case for Mn 2 Au. The susceptibility of Mn 2 Au is weak ( χ =5 × 10 −4 SI) and almost temperature independent above 50–100 K, which has been taken as a manifestation of Pauli paramagnetism [8] . However, from a first-principles Local Spin Density Approximation (LSDA) study, it was argued that Mn 2 Au should be AFM, with a large Mn magnetic moment, approaching 4 μ B per Mn, and a Néel temperature well above room temperature [9] . Subsequently, it was theoretically predicted that the Mn moments are confined in the basal plane of the tetragonal structure of this compound, with a sizeable in-plane anisotropy [3] . In this article, we provide an experimental confirmation of these theoretical predictions, therefore, establishing that Mn 2 Au is a particularly promising material for AFM spintronics. Magnetic susceptibility The temperature dependence of the experimental magnetization, M exp , measured under an applied field, μ 0 H app =1T, is shown in Fig. 1a . Above 100 K, the derived DC (direct current) susceptibility, χ exp (= M exp /H app ), is almost temperature independent, amounting to χ exp =5 × 10 −4 at 300 K. Below typically 100 K, an additional component develops, which is reminiscent of paramagnetic impurities. At low temperatures, a low-field nonlinear term is found for the variation of the magnetization, M exp , under field, obviously due to the same phenomenon leading to the low T increase in susceptibility. From 20 K to room temperature, the isotherm magnetization variation is essentially linear in field up to 7 T ( Fig. 1b ). At higher temperature, an up-turn starts to appear in the variation of the magnetization with applied field (see change of slope above 4 T at 400 K in Fig. 1b ). These results, which are in agreement with previous observations, will be analysed in the discussion section, after we have presented data from nuclear magnetic resonance (NMR) and neutron experiments concerning the magnetic structure of Mn 2 Au. 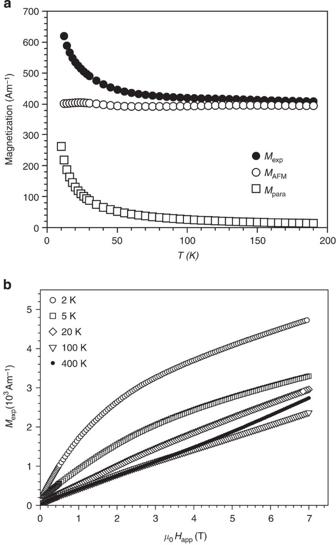Figure 1: Magnetic susceptibility measurements. (a) Filled circles: Temperature dependence of the experimental magnetization,Mexp, measured underμ0Happ=1 T. Squares: Calculated paramagnetic contribution to the magnetization of Mn moments located on Au sites,Mpara(see text). Open circles: Deduced magnetization,MAFM=Mexp−Mpara, representing the antiferromagnetic susceptibility under an applied magnetic fieldμ0Happ=1 T; (b) magnetization,Mexp, as a function of the applied magnetic field,μ0Happ, at temperaturesT=2, 5, 20, 100 and 400 K. Figure 1: Magnetic susceptibility measurements. ( a ) Filled circles: Temperature dependence of the experimental magnetization, M exp , measured under μ 0 H app =1 T. Squares: Calculated paramagnetic contribution to the magnetization of Mn moments located on Au sites, M para (see text). Open circles: Deduced magnetization, M AFM = M exp − M para , representing the antiferromagnetic susceptibility under an applied magnetic field μ 0 H app =1 T; ( b ) magnetization, M exp , as a function of the applied magnetic field, μ 0 H app , at temperatures T =2, 5, 20, 100 and 400 K. Full size image Nuclear magnetic resonance A 55 Mn zero-field nuclear magnetic resonance (NMR) spectrum, recorded at room temperature, reveals the existence of five absorption peaks in the frequency range, ν =186–195 MHz, as expected for the Zeeman levels of a spin I =5/2 shifted by the quadrupole interaction ( Fig. 2 ). The large intensity of the NMR signal shows that it is representative of the main Mn 2 Au phase and not of possible minority phases. Qualitatively, the presence of an NMR signal at such high frequencies in the absence of any external field demonstrates that 55 Mn nuclei experience a large hyperfine internal field, that is, Mn 2 Au is magnetically ordered at room temperature. The well-defined lines in the quadrupole-split spectrum and the absence of any additional spectral feature indicate that the spectrum can be modelled by a single site, in agreement with the single crystallographic site of Mn in Mn 2 Au: all Mn atoms experience the same hyperfine field, | H hyp |= ν / γ *=14.3 MA/m ( γ *= γ /2 π =10.55 MHzT −1 is the gyromagnetic ratio), and the same quadrupolar splitting of 0.9 MHz, without any distribution of angles between the principal axes of the magnetic hyperfine and electric field gradient tensors. The relatively large values, for a metallic sample at room temperature, of both the spin–lattice relaxation time T 1 (8 ms) and the spin–spin relaxation time T 2 (314 μs) suggest gapped spin excitations. This is consistent with magnetic order being well established at room temperature. 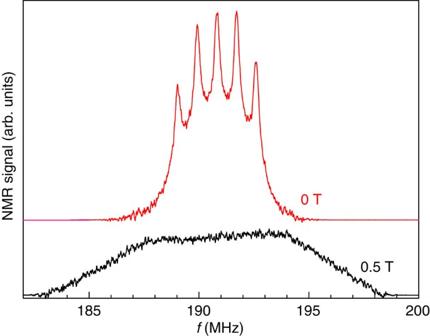Figure 2: Room temperature55Mn NMR spectra of Mn2Au. In red: zero-field spectrum. In black: spectrum underμ0Happ=0.5 T. Figure 2: Room temperature 55 Mn NMR spectra of Mn 2 Au. In red: zero-field spectrum. In black: spectrum under μ 0 H app =0.5 T. Full size image Applying a magnetic field of μ 0 H app =0.5 T changes the five-peak spectrum observed in zero-field into an unresolved broad spectrum extending from 183 to 198 MHz ( Fig. 2 ). This effect is typical of AFM systems for which the equivalence of all sites in the constituent grains breaks down with the appearance of a distribution of angles between internal and applied fields [10] . The total field experienced by 55 Mn nuclei takes all values between H hyp + H app and − H hyp + H app , which explains the additional extension of the spectrum by ~4 MHz in both directions. Magnetic structure determination using neutron diffraction In order to determine the exact magnetic structure of Mn 2 Au, a neutron diffraction study was performed on the D1B diffractometer at the Institut Laue-Langevin (Grenoble, France). A neutron wavelength of 1.28 Å was used. Below 900 K, the main peaks of all diffraction patterns are characteristic of the Mn 2 Au phase (2 K pattern shown in Fig. 3 ). Small additional peaks are present that can be associated with (i) the nuclear and magnetic peaks of MnAu, which orders antiferromagnetically ( k =0 ½ 0) at T N =523 K, and (ii) a small MnO impurity, not visible in the laboratory X-ray data (method section), having the AFM structure ( k =½ ½ ½) at T N =118 K. Quantitative Rietveld analysis [11] of the neutron data gave a value of 2.3 weight % MnAu, in excellent agreement with the value derived from X-ray data. The MnO impurity phase amounted to 0.4(1)% (see Fig. 3 and Supplementary Fig. S1 ). The 2 K pattern was initially analysed under the assumption that no magnetism is present in Mn 2 Au, that is, only nuclear scattering is involved ( Fig. 4a ). The diagram calculated within FULPROF displays all experimentally observed reflections [11] . However, at low scattering angles, the experimental intensities of almost all reflections are larger than the calculated ones, and the discrepancy may be larger than the statistical error by up to three orders of magnitude. This suggests the existence of magnetic contributions to the Bragg reflections, with a magnetic structure described in the same cell as the crystallographic one, that is, a propagation vector equal to [000]. This type of order may be described as an intra-unit cell AFM order. The neutron diffraction pattern was thus compared with each of the patterns expected for the magnetic structures allowed by the group theory within the tetragonal structure of Mn 2 Au. The representational analysis followed the formalism of Bertaut [12] , with the SARA h [13] http://www.ccp14.ac.uk , SARAh (2000) programme. The representations were constructed with the m k Fourier components corresponding to the Mn atoms at the 4 e position (0, 0, z). The different basis vectors, which are associated with each irreducible representation, were also calculated. Table 1 gives the four possible magnetic structures, consistent with I 4/mmm symmetry and k =[000], together with the resulting magnetic space group. Two possible magnetic structures, Γ3 and Γ9, can be discarded, as they are ferromagnetic. The two AFM structures (Γ2 and Γ10) were carefully examined. The fit corresponding to the Γ2 structure is shown in Fig. 4b , whereas the one corresponding to Γ10 is shown in Fig. 3 . Only the latter is compatible with the experimental data and it corresponds to the [ A x , A y , 0] basis functions. The resulting magnetic space group is Im'mm. The Mn moments, μ Mn , form ferromagnetic sheets perpendicular to c . Their orientation alternates from one sheet to the next. This structure is identical to that theoretically predicted by Khmelevskyi and Mohn [9] . The moments are confined in the plane perpendicular to the uniaxial axis, c , in agreement with the large intensity of the 00l reflections. Due to the tetragonal symmetry of the Mn 2 Au crystallographic structure, the neutron analysis does not allow the determination of the direction of the moments within the plane. In the scheme of Fig. 5 , the moments within the (001) plane are arbitrarily represented along the [110] basal plane direction (see below). At 2 K, the Mn atoms bear a moment of 4.0(3) μ B . The refinement converged to a magnetic R -factor value of 2.63. In the whole temperature range, from 2 to 900 K, the analysis provides essentially the same result ( Supplementary Table S2 ). The temperature dependence of the Mn magnetic moment in the whole range of measured temperatures is remarkably weak ( Fig. 6 ). At the highest temperature (900 K), the Mn moment still amounts to approximately 85% of its value at 0 K. Note that the value of the Mn moment in the analysis is strongly correlated to the value of the B thermal factors. At room temperature, the thermal factors of Au and Mn were fixed at values identical to those determined by X-ray diffraction ( B iso in Supplementary Table S1 ). At the other temperatures, an overall additional B factor was refined (noted B ov in Supplementary Table S2 ). 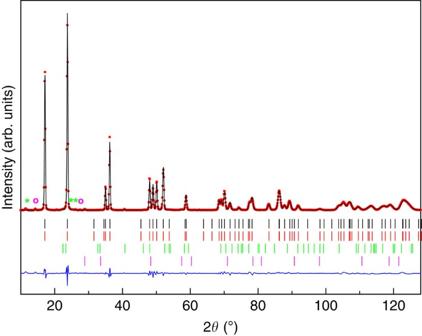Figure 3: Mn2Au neutron diffraction pattern recorded at 2 K and optimum fit obtained. Red: experimental data, black: fit to the data corresponding to the Γ10 magnetic structure, faint black line in the lower part of the figure: difference between experiment and fit. Another antiferromagnetic structure is compatible with the group theory, noted Γ2 (seeTable 1), but it is incompatible with experimental data (Fig. 4b). Black and red ticks: nuclear and magnetic diffraction peaks of Mn2Au; green ticks: nuclear diffraction peaks revealing the presence of AuMn (impurity amounting to 2.3% of the total sample according to quantitative Rietveld analysis); purple ticks: nuclear diffraction peaks revealing the presence of MnO (impurity amounting to 0.4% of the total sample); green stars: magnetic diffraction peaks associated with the MnAu impurity; purple circles: magnetic diffraction peaks associated with the MnO impurity. Figure 3: Mn 2 Au neutron diffraction pattern recorded at 2 K and optimum fit obtained. Red: experimental data, black: fit to the data corresponding to the Γ10 magnetic structure, faint black line in the lower part of the figure: difference between experiment and fit. Another antiferromagnetic structure is compatible with the group theory, noted Γ2 (see Table 1 ), but it is incompatible with experimental data ( Fig. 4b ). Black and red ticks: nuclear and magnetic diffraction peaks of Mn 2 Au; green ticks: nuclear diffraction peaks revealing the presence of AuMn (impurity amounting to 2.3% of the total sample according to quantitative Rietveld analysis); purple ticks: nuclear diffraction peaks revealing the presence of MnO (impurity amounting to 0.4% of the total sample); green stars: magnetic diffraction peaks associated with the MnAu impurity; purple circles: magnetic diffraction peaks associated with the MnO impurity. 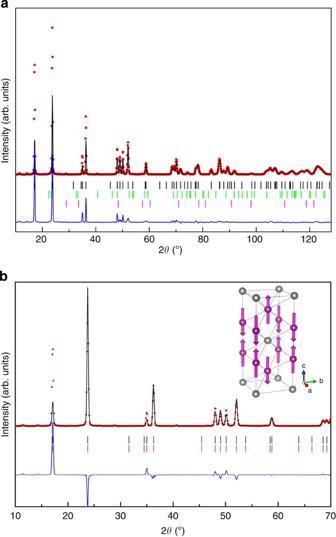Figure 4: Other tentative fits to the 2 K neutron diffraction pattern of Mn2Au. (a) Assuming only nuclear scattering; red: experimental data, black: fit to the data assuming only nuclear scattering. The discrepancy (difference pattern in blue) between observed and calculated intensities may reach orders of magnitude. (b) Expected for the antiferromagnetic Γ2 structure; red: experimental data, black: fit to the data, blue: difference between experiment and fit. The large discrepancy at low scattering angles establishes that Γ2 cannot be the real magnetic structure of Mn2Au. Inset: schematic representation of the Γ2 magnetic structure. Full size image Figure 4: Other tentative fits to the 2 K neutron diffraction pattern of Mn 2 Au. ( a ) Assuming only nuclear scattering; red: experimental data, black: fit to the data assuming only nuclear scattering. The discrepancy (difference pattern in blue) between observed and calculated intensities may reach orders of magnitude. ( b ) Expected for the antiferromagnetic Γ2 structure; red: experimental data, black: fit to the data, blue: difference between experiment and fit. The large discrepancy at low scattering angles establishes that Γ2 cannot be the real magnetic structure of Mn 2 Au. Inset: schematic representation of the Γ2 magnetic structure. Full size image Table 1 Possible magnetic structures for Mn 2 Au. 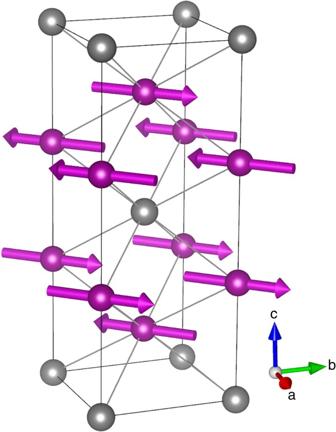Figure 5: Magnetic structure of Mn2Au derived from the neutron diffraction study. The Mn moments form ferromagnetic sheets perpendicular toc. Their orientation alternates from one sheet to the next. The moments are confined in the plane perpendicular to the uniaxial axis,c. The neutron analysis does not allow the determination of the direction of the moments within the plane. Full size table Figure 5: Magnetic structure of Mn 2 Au derived from the neutron diffraction study. The Mn moments form ferromagnetic sheets perpendicular to c . Their orientation alternates from one sheet to the next. The moments are confined in the plane perpendicular to the uniaxial axis, c . The neutron analysis does not allow the determination of the direction of the moments within the plane. 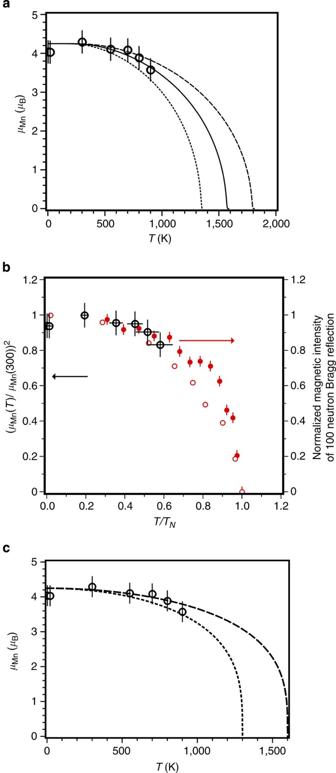Figure 6: Temperature dependence of the Mn magnetic moment. (a) Temperature dependence of the Mn magnetic moment compared with dependences given by the Brillouin functionS=2. Open black dots: experimental Mn magnetic moment derived from the neutron data (The vertical bars are the errors obtained in the quantitative Rietveld analysis of the neutron data.). Calculated temperature dependences forTN=1,575 K (continuous line),TN=1,350 K (dotted line) andTN=1,800 K (dashed line). (b) Comparison of the temperature dependence of neutron magnetic intensities in Mn2Au with temperature dependences found in other antiferromagnetic systems. Open black dots: square of the Mn magnetic moment in Mn2Au (left scale). The point positions correspond toTN=1,450 K, whereas the two extremes of the horizontal error bars correspond toTN=1,300 K andTN=1,600 K, respectively. In red:T/TNdependence of the normalized magnetic intensity of the 100 Bragg reflection (expected to be proportional to the square of the Mn magnetic moment) in antiferromagnetic Mn3Ir (filled circles)14and MnPd (open circles)15. (c) Comparisons of the temperature dependence of the Mn magnetic moment in Mn2Au with the temperature dependence predicted for the phenomenological expression(see text). Open black dots: Mn magnetic moment. Calculated temperature dependences of the Mn magnetic moment obtained forα=2,β=0.3 and two different assumed values ofTN=1,300 K (dotted line) and 1,600 K (dashed line), respectively. Full size image Figure 6: Temperature dependence of the Mn magnetic moment. ( a ) Temperature dependence of the Mn magnetic moment compared with dependences given by the Brillouin function S =2. Open black dots: experimental Mn magnetic moment derived from the neutron data (The vertical bars are the errors obtained in the quantitative Rietveld analysis of the neutron data.). Calculated temperature dependences for T N =1,575 K (continuous line), T N =1,350 K (dotted line) and T N =1,800 K (dashed line). ( b ) Comparison of the temperature dependence of neutron magnetic intensities in Mn 2 Au with temperature dependences found in other antiferromagnetic systems. Open black dots: square of the Mn magnetic moment in Mn 2 Au (left scale). The point positions correspond to T N =1,450 K, whereas the two extremes of the horizontal error bars correspond to T N =1,300 K and T N =1,600 K, respectively. In red: T / T N dependence of the normalized magnetic intensity of the 100 Bragg reflection (expected to be proportional to the square of the Mn magnetic moment) in antiferromagnetic Mn 3 Ir (filled circles) [14] and MnPd (open circles) [15] . ( c ) Comparisons of the temperature dependence of the Mn magnetic moment in Mn 2 Au with the temperature dependence predicted for the phenomenological expression (see text). Open black dots: Mn magnetic moment. Calculated temperature dependences of the Mn magnetic moment obtained for α =2, β =0.3 and two different assumed values of T N =1,300 K (dotted line) and 1,600 K (dashed line), respectively. Full size image Assuming that the temperature dependence of the Mn moment corresponds to that given by the S =2 Brillouin function, a Néel temperature of 1575 (225) K is extrapolated from the present data (see Fig. 6a ). As mean field models tend to overestimate magnetic ordering temperatures, this value can be seen as an upper limit for the Néel temperature of Mn 2 Au. To obtain a more reliable value of T N, , the experimentally determined temperature dependence of the Mn sub-lattice moment in Mn 2 Au was compared with the temperature dependence found in other AFM Mn compounds with Néel temperatures well above room temperature, namely Mn 3 Ir ( T N =960 K) [14] and MnPd ( T N =535 K) [15] . For these two compounds, the T / T N dependence of the reduced intensity of the 100 magnetic Bragg reflection (proportional to the square of the magnetic moment), as measured by neutron diffraction, is shown in Fig. 6b . The value of T N in Mn 2 Au was adjusted so that the T / T N dependence of the square of the Mn magnetic moment resembles those found for Mn 3 Ir and MnPd. Under such an hypothesis, the T N value of Mn 2 Au is found to be in the temperature interval 1,300–1,600 K. Furthermore, the experimental temperature dependence of the sub-lattice Mn moment, μ Mn ( T ), in Mn 2 Au was calculated according to the phenomenological expression [16] : where α and β are parameters. At low temperature, the moment varies as 1− cT α , whereas close to T N it varies as [1−( T / T N ) β ] (Kuz’min [17] proposed a similar expression to describe the temperature dependence of the spontaneous magnetization in ferromagnetic systems). The parameter values α =2 and β =0.3 were taken, corresponding to average values derived from fits of the temperature dependence of neutron intensities in Mn 3 Ir and MnPd. Note that α =2 is the exponent predicted by spin-wave theory in antiferromagnets and β =0.3 is close to the 3D Heisenberg critical exponent of 0.33. The, thus, calculated temperature dependence of the manganese moment is compared with the experimental data in Fig. 6c , for T N equal to 1,300 and 1,600 K, respectively. The ratio between the Mn magnetic moment value, as deduced from neutron scattering, and the hyperfine field measured by NMR on 55 Mn gives a hyperfine coupling constant of 5.5 Tμ B −1 . In Mn compounds where the on-site contribution to the hyperfine field dominates, the hyperfine coupling constant is usually of the order of 10–15 Tμ B −1 (ref. 18 ). The low value found in Mn 2 Au might be attributed to a transferred hyperfine field from the nearest Mn neighbours, having a sign opposite to the dominant on-site contribution. Such a large transferred hyperfine field has been found in a number of R-Mn compounds (R=rare-earth) [19] . Not only is the magnetic structure of Mn 2 Au determined in this study identical to that predicted by first-principles calculations, but also, the value of the Mn magnetic moment, 4.0 (3) μ B at 2 K, is consistent with the calculated value of 3.64 μ B and the Néel temperature, evaluated to be in the range of 1,300–1,600 K, which is compatible with the theoretical value of 1,610 K (ref. 9 ). Introducing SO coupling in a self-consistent second-variational procedure, the magnetocrystalline anisotropy may be evaluated at 0 K using the torque method [3] . It amounts to −25 K per Mn 2 Au (corresponding to a second-order anisotropy constant K =7.3 × 10 6 J m −3 ), where the negative sign means that the basal plane is favoured with respect to the uniaxial axis. Among metallic AFM alloys, Mn-Ir close to the 3:1 composition is known to have a large magnetocrystalline anisotropy. From the analysis of the blocking temperature of Mn-Ir nanograins, O’Grady et al. [20] have derived that the room temperature second-order anisotropy constant is of the order of 5.5 × 10 5 J m −3 . In order to evaluate the room temperature anisotropy in Mn 2 Au, one may use the approximate Akulov expression [21] , according to which the anisotropy coefficients of order l should vary with temperature as , where m is the reduced magnetization. Introducing in this expression the temperature dependence of the sub-lattice magnetization given by Equation (1) above, one derives that the second-order anisotropy coefficient at 300 K is of the order of 90% of the 0 K value. The anisotropy in Mn 2 Au is thus expected to be at least an order of magnitude higher than in Mn-Ir. Although not providing a quantitative value for the anisotropy energy, the neutron study is consistent with calculations, in establishing that the Mn moments are in the basal plane of the tetragonal structure. The in-plane fourth-order anisotropy of Mn 2 Au is evaluated below. It is much weaker than the here-discussed second-order anisotropy and this constitutes an important element for TAMR. Having established the existence of an AFM order in Mn 2 Au with NMR and neutron studies, we will now analyse the magnetic susceptibility of Fig. 1 within the molecular field model. The magnetic energy, E m , may be expressed as: where N =42 × 10 27 m −3 is the number of Mn atoms per unit volume, M sl is the Mn sublattice magnetization, W is the coefficient representing interactions within a given AFM sublattice and W ′ is the coefficient representing interactions between sublattices. The perpendicular susceptibility, , is equal to 1/ W ′. For an isotropic powdered sample, the low-T susceptibility, χ , should be equal to 2/3 . From χ =5 × 10 −4 SI and M sl =0.78 × 10 6 A m −1 (corresponding to 4 μ B per Mn), one derives W′ =1,330. We have no experimental means to evaluate W . The values of the three principal exchange integrals (see Fig. 1 in ref. 9 ): J 1 ( J 1 k B −1 =−396 K) and J 2 ( J 2 k B −1 =−532 K) (representing coupling with Mn moments in the other sub-lattice) and J 3 ( J 3 k B −1 =115 K) (characterizing the interaction within a given sub-lattice) were derived in the already mentioned first-principle calculations [9] . Term to term identification gives: μ 0 W ′ M sl 2 = N (4 J 1 + J 2 ) k B and μ 0 W M sl 2 = N × 4 J 3 k B . Assuming that the ratio between the W values is identical to that derived from the theoretical calculations, gives W =290. The Néel temperature then derived from equation (2) amounts to 1,435 (200) K, a value in agreement with the one derived from the neutron analysis. In AFM materials, a spin-flop transition may be observed at a field, , where H exch = W ′ M sl ( μ 0 H exch =1,300 T in Mn 2 Au, derived from susceptibility measurements) is the intersublattice exchange field and H A = K / μ 0 M sl ( μ 0 H A =10 T in Mn 2 Au, derived from theoretical second-order anisotropy) is the anisotropy field. At H sf , a change in the magnetic susceptibility occurs. In the present case, the spin-flop transition is predicted to occur at H sf =123 × 10 6 A m −1 ( μ 0 H sf =150 T), a value beyond possible experimental observation. As the Mn moments are confined in the basal plane of the structure, another spin-flop transition may occur due to the in-plane fourth-order anisotropy (difference in energy between the [100] and [110] directions). Attributing to this phenomenon, the change in susceptibility under μ 0 H app =5 T at T =400 K ( Fig. 1b ), an in-plane anisotropy field of approximately μ 0 H A =0.01 T is deduced. In ref. 3 , the calculated 0 K in-plane anisotropy field amounts to 0.04 T. Applying the law for l =4, gives approximately 0.03 T at 400 K, which is of the order of the experimentally determined value. This low in-plane anisotropy energy indicates that TAMR structures based on Mn 2 Au could exploit the in-plane rotation of the Mn moments from one easy in-plane direction to the other [3] . The susceptibility increase found in the present study below around 100 K, as well as in the initial study of Mn 2 Au [8] , may be attributed to ‘impurity’ Mn atoms occupying the Au site [9] . The exchange coupling on these Mn moments is zero, the different contributions cancelling each other out. χ para , the contribution of such paramagnetic uncoupled moments to the total susceptibility χ exp , was calculated assuming an effective Mn moment of 4.9 μ B (derived from S =2, in agreement with the low-temperature 4 μ B Mn moment). The fraction x of Au sites occupied by Mn atoms was determined by imposing that the susceptibility, χ AFM = χ exp − χ para , be approximately constant, as expected for an antiferromagnet at low-T (see Fig. 1a , note that in this figure the magnetization in A m −1 under 1 T is plotted and not the susceptibility, thus the notation M exp , M para and M AFM ). The obtained value of x is 0.25% (the exchange-field on the Mn impurity moments due to the canting under field of the normal Mn moments was neglected). This very small value indicates that the atomic order in Mn 2 Au is close to perfect. Mn atoms on the Au sites would inevitably introduce undesired frustration. The high value of the Néel temperature in Mn 2 Au and the fact that it is close to the theoretical value are additional indications of the quality of the atomic order in this compound. Ten-nanometre-thick films of Mn 2 Au have recently been prepared by molecular beam epitaxy, on top of a 5-nm-thick Fe film, itself grown on (001) MgO (ref. 5 ). The observation of exchange-bias behaviour provided convincing but indirect evidence of AFM order in Mn 2 Au. The present study establishes the AFM nature of this compound unambiguously. The experimentally determined magnetic structure is identical to that theoretically predicted. The Néel temperature is found to be between 1,300 K and 1,600 K, which should be compared with 1,145 K in MnIr and below 500 K in recently discovered CuMnAs (ref. 4 ). Large magnetoresistance anisotropy requires large SO coupling effects, which, in a uniaxial structure, may lead to the existence of a large magnetocrystalline anisotropy. In case the magnetic moments align along the unique axis, the difficulty in rotating them from the easy axis to the basal plane makes it impossible to exploit TAMR effects. In Mn 2 Au, on the contrary, the moments being in the basal plane of the structure, their rotation from one easy in-plane direction to the other may be obtained under the effect of a relatively small external excitation (for example, by coupling to an external applied field, involving the exchange-spring phenomenon as in MnIr(ref. 6 )). This provides the mechanism for large TAMR effects as illustrated in Fig. 7 . In the absence of SO interactions, the Mn orbitals would take the fourfold basal plane symmetry of the tetragonal structure ( Fig. 7a ). However, owing to the strong SO coupling resulting from Mn-Au hybridization, the Mn orbitals take a uniaxial symmetry, the principal axis of the electron distribution becoming the moment direction ( Fig. 7b,c ). Assume a TAMR stack made of two Mn 2 Au layers separated by an insulating barrier, the moment direction in one layer being fixed, as in Fig. 7b , for example, whereas in the other it may rotate from (b) to (c). Owing to the anisotropy in interfacial hybridization, the tunnel current will depend on whether the directions of the AFM moments are the same in both layers or arranged at 90° to each other. 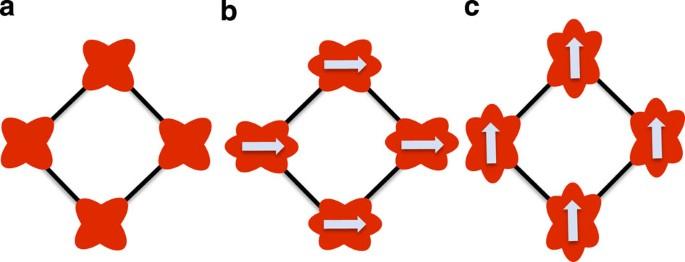Figure 7: Illustration of the mechanism by which low-field large TAMR may be expected in Mn2Au. (a) In the absence of spin-orbit interactions, the Mn orbitals (in red) take the fourfold basal plane symmetry of the tetragonal structure. (b,c) Under the influence of spin-orbit coupling, the Mn orbitals take a uniaxial symmetry, the principal axis of the electron distribution becoming the moment direction. Owing to anisotropy in interfacial hybridization, the tunnel current, in a stack made of two Mn2Au layers separated by a tunnel barrier, will depend on whether the directions of the AFM moments are identical (b-borc-c) or perpendicular (b-c). Figure 7: Illustration of the mechanism by which low-field large TAMR may be expected in Mn 2 Au. ( a ) In the absence of spin-orbit interactions, the Mn orbitals (in red) take the fourfold basal plane symmetry of the tetragonal structure. ( b , c ) Under the influence of spin-orbit coupling, the Mn orbitals take a uniaxial symmetry, the principal axis of the electron distribution becoming the moment direction. Owing to anisotropy in interfacial hybridization, the tunnel current, in a stack made of two Mn 2 Au layers separated by a tunnel barrier, will depend on whether the directions of the AFM moments are identical ( b - b or c - c ) or perpendicular ( b - c ). Full size image In all TAMR structures developed to date, the tunnel magnetoresistance was found to decrease rapidly with increasing temperature and this was tentatively related to the degradation of the ordered magnetic state, which is the source of the TAMR signal [2] , [6] . The large exchange interactions required to preserve close-to-ground-state properties above room temperature, are present in Mn 2 Au, which is among the materials having the highest magnetic ordering temperature. Mn 2 Au appears to optimally combine all the required properties for becoming a cornerstone of future AFM spintronic devices. Sample preparation and characterization An ingot of Mn 2 Au was prepared by induction melting and annealed for 3 days at 650 °C, below the peritectic temperature of 680 °C, at which the Mn 2 Au phase decomposes. The annealed sample was ground into powder with a typical particle size of 5 μm and, after being sealed in a quartz tube, it was annealed at 350 °C for 1 h to remove strain induced by grinding. X-ray diffraction A detailed X-ray diffraction pattern was taken using Cu radiation ( λ Cu =1.54 Å). An excellent fit to the known MoSi 2 -type tetragonal structure of Mn 2 Au was obtained using Rietveld analysis (FULPROF software; Supplementary Table S1 ) [11] . Impurity reflections were detected, arising from MnAu. The weight fraction of MnAu in the sample, derived from quantitative phase analysis of the diffraction pattern, is 2.5(4)%. The possible occupancy of Au sites by Mn atoms converged to a value of 3 (3)%, of which the difference from zero is not statistically significant. Magnetometry The DC susceptibility was measured using a Quantum Design VSM-SQUID, in fields up to 7 T and in the temperature range of 2–400 K. Two types of measurements were performed, either with the Mn 2 Au powder free in the sample holder or embedded in an epoxy resin. Both types of measurements gave identical results. NMR The NMR experiment was performed on a home-built heterodyne spectrometer using standard spin-echo techniques. The frequency was scanned between 80 and 275 MHz. The 55 Mn spectrum was obtained by combining Fourier transforms of the spin-echo signal recorded for regularly spaced frequency values. Neutron diffraction The neutron diffraction study was performed on the D1B diffractometer at the Institut Laue-Langevin (Grenoble, France). A neutron wavelength of 1.28 Å was used. At this wavelength, the neutron flux is eight times less intense than at 2.52 Å. However, the Ewald sphere contains a larger volume of the reciprocal space and there is no λ /2 contamination. Neutron diffraction patterns were recorded at temperatures T =2, 20, 300 550 700, 800 and 900 K. The neutron diffraction pattern recorded at 2 K revealed that two main impurities are present in the sample: MnAu amounting to 2.3% of the total sample and MnO amounting to 0.4% (see Supplementary Fig. S1 ). The 2 K pattern was initially analysed under the assumption that no magnetism is present in Mn 2 Au, that is, only nuclear scattering is involved ( Fig. 4a ). The diagram calculated within FULPROF displays all experimentally observed reflections [11] . However, at low scattering angles, the experimental intensities of almost all reflections are larger than the calculated ones, and the discrepancy may be larger than the statistical error by up to three orders of magnitude. This suggests the existence of magnetic contributions to the Bragg reflections, with a magnetic structure described in the same cell as the crystallographic one, that is, a propagation vector equal to [000]. The neutron diffraction pattern was thus compared with each of the patterns expected for the magnetic structures allowed by group theory within the tetragonal structure of Mn 2 Au. Of these, two are AFM (Γ2 and Γ10) and they were carefully examined. The fit corresponding to the Γ2 structure is shown in Fig. 4b (the structure is shown in the inset), whereas the one corresponding to Γ10 is shown in Fig. 3 . Only the latter structure (Γ10) is compatible with the experimental data. The high-temperature transformation of Mn 2 Au into MnAu and γ-Mn was followed by collecting a series of short-duration neutron diffraction patterns, as the sample was slowly heated from 900 to 1,000 K. This is not of direct relevance for the present study and is not described in further detail in this paper. How to cite this article: Barthem, V.M.T.S. et al. Revealing the properties of Mn 2 Au for antiferromagnetic spintronics. Nat. Commun. 4:2892 doi: 10.1038/ncomms3892 (2013).